MicroRNA-431 accelerates muscle regeneration and ameliorates muscular dystrophy by targeting Pax7 in mice Skeletal muscle stem cells, called satellite cells, are a quiescent heterogeneous population. Their heterogeneity is influenced by Pax7, a well-defined transcriptional regulator of satellite cell functions that defines two subpopulations: Pax7 Hi and Pax7 Lo . However, the mechanisms by which these subpopulations are established and maintained during myogenesis are not completely understood. Here we show that miR-431, which is predominantly expressed in the skeletal muscle, mediates satellite cell heterogeneity by fine-tuning Pax7 levels during muscle development and regeneration. In miR-431 transgenic mice, the Pax7 Lo subpopulation is enriched, enhances myogenic differentiation and accelerates muscle regeneration. Notably, miR-431 attenuates the muscular dystrophic phenotype in mdx mice and may be a potential therapeutic target in muscular diseases. miR-431 transgenic mice are a unique genetic model for investigating the cellular features and biological functions of Pax7 Lo satellite cells during muscle development and regeneration. Adult skeletal muscle has a remarkable regenerative capacity that is attributable to satellite cells (SCs), which express the paired-box transcriptional factor Pax7 (refs 1 , 2 , 3 , 4 ). In resting muscle, SCs are mostly quiescent; however, in response to stress or injury, they become activated and proliferated and either undergo differentiation or self-renewal to replenish the quiescent cell pool [5] , [6] , [7] , [8] . During regeneration, skeletal muscle must strike a delicate balance between differentiation and self-renewal to maintain SC homeostasis [9] . This process is tightly regulated by extrinsic cues, namely by various factors in the stem-cell niche and by intrinsic transcriptional regulators, including Pax7, Myf5 and MyoD [4] , [6] , [10] , [11] , [12] . Pax7 contributes to SC activation, proliferation, self-renewal and differentiation by regulating expression of its target genes, such as Myf5 and MyoD [13] , [14] . Pax7 is critical for the development and regeneration of skeletal muscles. In Pax7 knockout mice, the SC lineage is progressively lost through defective proliferation and self-renewal and precocious differentiation [1] , [4] , [10] , [15] . Pax7 also helps to direct and maintain the lineage specification of SCs, which in the absence of Pax7 and Pax3 differentiate into cartilage and other nonmuscle cell types [16] . Importantly, Pax7 +/+ cells are essential for adult skeletal muscle regeneration after skeletal muscle injury [17] . More intriguingly, SCs are highly heterogeneous [18] , [19] , and recent studies have shown that different levels of Pax7 expression produce two subpopulations of SCs—Pax7 Hi and Pax7 Lo —that have distinct biological features in mice [20] . Pax7 Lo cells are primed more for myogenic differentiation and less for self-renewal and higher metabolic status than Pax7 Hi cells. It is unclear which signals establish and maintain SC heterogeneity. Precise control of Pax7 levels is critical for its function in mediating SC heterogeneity [20] . During development and adult skeletal muscle regeneration, regulation of Pax7 expression is tightly correlated with SC function. Pax7 is expressed abundantly in quiescent SCs but at much lower levels in activated SCs. Furthermore, Pax7 downregulation is required for myogenic differentiation [21] . However, the mechanism that governs Pax7 expression in SCs during muscle development and regeneration is unclear. A better understanding of this mechanism might help to reveal how Pax7 Hi and Pax7 Lo subpopulations are established and maintained. MicroRNAs (miRNAs) help to regulate many cellular processes, including cell-fate determination, proliferation, differentiation and apoptosis, by refining gene expression at the transcriptional or post-transcriptional level [22] , [23] , [24] , [25] , [26] . Particularly, knocking out Dicer (an RNase III endonuclease responsible for miRNA maturation) in mouse skeletal muscle with MyoD-Cre or Pax7-Cre showed that many miRNAs are required for muscle development and SC functions [27] , [28] . For example, miR-1 and miR-133 are induced during skeletal muscle differentiation and are the key regulators of myoblast proliferation and differentiation [29] . miR-1 and miR-206 regulate SC differentiation by repressing Pax7 (ref. 30 ). miR-27a, which is expressed in differentiating skeletal muscle of the embryonic myotome and is activated in SCs of adult muscles, promotes SC differentiation by targeting Pax3 (ref. 31 ). miR-489, which is highly expressed in quiescent SCs and is quickly downregulated during SC activation, helps to maintain the quiescent state of adult stem-cell populations by targeting Dek [27] . When miRNA expression in skeletal muscle is dysregulated, various skeletal muscle disorders ensue, including skeletal muscle hypertrophy and muscular dystrophy [32] , [33] , [34] . Since Pax7 levels affect the heterogeneity of SCs and define two subpopulations, Pax7 Hi and Pax7 Lo , and miRNAs help to fine-tune post-translational gene expression, we hypothesized that miRNA helps to establish and maintain these subpopulations by precisely modulating Pax7 levels. Here we describe the identification and characterization of miR-431, which is predominantly expressed in skeletal muscle tissue and regulates myogenic differentiation. We find that miR-431 mediates satellite-cell heterogeneity during muscle development and regeneration by targeting Pax7 . Skeletal muscle-expressed miR-431 directly targets Pax7 To identify miRNAs important for fine-tuning Pax7 levels, we searched for potential miRNA-binding sites in the 3′-untranslated repeat (UTR) of Pax7 mRNA with TargetScan and miRanda. miR-431 ( Supplementary Fig. 1 ) has two such binding sites ( Fig. 1a ) and resides within the miRNA cluster opposite to the orientation of the retrotransposon-like 1 ( Rtl1 ) gene in the Dlk1-Dio3 region ( Supplementary Fig. 2 ). miR-431 is predominantly expressed in mouse skeletal muscle ( Fig. 1b ). During the rapid growth that occurs during the first 3 weeks of postnatal myogenesis, miR-431 is highly expressed ( Supplementary Fig. 3 ). During in vitro differentiation of isolated SCs, miR-431 expression increases gradually ( Fig. 1c ); in parallel, Pax7 expression decreases ( Fig. 1d ). Moreover, we examined expression of Pax7 and miR-431 in freshly isolated myoblasts from muscle in postnatal 3-week pups (SC in proliferating state) and 12-week adult mice (SC in quiescence). Pax7 expression was significantly lower in 3- than in 12-week-old myoblasts; conversely, miR-431 was expressed at significantly higher levels in isolated myoblasts from 3-week-old mice than that from 12-week-old mice ( Supplementary Fig. 4 ). Together, the unique expression pattern of miR-431 and its binding sites at the 3′-UTR of Pax7 mRNA suggests that miR-431 regulates myogenesis by targeting Pax7 . 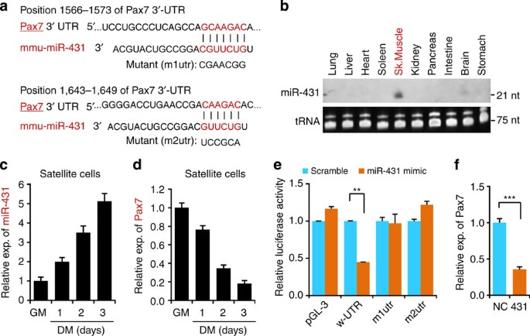Figure 1: miR-431 is predominantly expressed in the skeletal muscle and targetsPax7in myogenic cells. (a) miR-431 target sequence alignment in thePax73′-UTR predicted with TargetScan. Two predicted target sites of miR-431 in the 3′-UTR of mousePax7are shown. The nucleotide coordinate ofPax7was based on the mouse Refseq (NM_011039). m1utr and m2utr, mutated from the seed matches, are indicated. (b) Expression of miR-431 in tissues from 3-week-old mice was analysed using northern blot analysis. Total RNA (20 μg) was loaded to detect miR-431, and tRNA was used as a loading control. (c,d) Expression of miR-431 andPax7during satellite cell proliferation (growth medium; GM) and differentiation (differentiation medium; DM) was assayed using real-time RT–qPCR. U6 small nuclear RNA (snRNA) served as an internal control for miR-431 expression, andGAPDHas a control forPax7detection. exp, expression. (e) Effect of miR-431 transfection in HEK 293 cells, measured with luciferase assays. Empty pGL-3 vector was a negative control. w-UTR is aPax7-3′-UTR, with miR-431-binding site inserted downstream of the luciferase gene in the pGL-3 control vector. m1utr and m2utr are mutant forms of thePax73′-UTR. A Renilla luciferase plasmid was co-transfected with a firefly luciferase construct as a transfection control. The results are expressed as firefly luciferase activity relative to Renilla luciferase activity. Values are means±s.e.m. of three independent measurements. **P<0.01. (f) miR-431 was overexpressed in C2C12 cells with a lentiviral system. Cells stably expressing a scramble sequences served as negative controls (NC).Pax7expression was determined using RT–qPCR. Error bars represent means±s.e.m. of three independent experiments. ***P<0.001. Two-tailed Student’st-test was used for all statistical testings. Figure 1: miR-431 is predominantly expressed in the skeletal muscle and targets Pax7 in myogenic cells. ( a ) miR-431 target sequence alignment in the Pax7 3′-UTR predicted with TargetScan. Two predicted target sites of miR-431 in the 3′-UTR of mouse Pax7 are shown. The nucleotide coordinate of Pax7 was based on the mouse Refseq (NM_011039). m1utr and m2utr, mutated from the seed matches, are indicated. ( b ) Expression of miR-431 in tissues from 3-week-old mice was analysed using northern blot analysis. Total RNA (20 μg) was loaded to detect miR-431, and tRNA was used as a loading control. ( c,d ) Expression of miR-431 and Pax7 during satellite cell proliferation (growth medium; GM) and differentiation (differentiation medium; DM) was assayed using real-time RT–qPCR. U6 small nuclear RNA (snRNA) served as an internal control for miR-431 expression, and GAPDH as a control for Pax7 detection. exp, expression. ( e ) Effect of miR-431 transfection in HEK 293 cells, measured with luciferase assays. Empty pGL-3 vector was a negative control. w-UTR is a Pax7 -3′-UTR, with miR-431-binding site inserted downstream of the luciferase gene in the pGL-3 control vector. m1utr and m2utr are mutant forms of the Pax7 3′-UTR. A Renilla luciferase plasmid was co-transfected with a firefly luciferase construct as a transfection control. The results are expressed as firefly luciferase activity relative to Renilla luciferase activity. Values are means±s.e.m. of three independent measurements. ** P <0.01. ( f ) miR-431 was overexpressed in C2C12 cells with a lentiviral system. Cells stably expressing a scramble sequences served as negative controls (NC). Pax7 expression was determined using RT–qPCR. Error bars represent means±s.e.m. of three independent experiments. *** P <0.001. Two-tailed Student’s t -test was used for all statistical testings. Full size image To directly validate Pax7 as a target of miR-431, we used a luciferase reporter construct containing a partial sequence of the Pax7 -3′-UTR encompassing two miR-431-binding sites. Co-transfection of HEK 293 cells with miR-431 and the wild-type (WT) 3′-UTR of Pax7 (w-UTR) repressed luciferase activity ( Fig. 1e ). This repression was abolished by co-transfection with miR-431 and reporters containing mutant forms of the miR-431-binding sites on Pax7 (m1utr or m2utr; Fig. 1e ). In C2C12 cells overexpressing miR-431, endogenous Pax7 mRNA levels were markedly reduced ( Fig. 1f ), confirming that miR-431 directly targets Pax7 . miR-431 promotes myogenic differentiation by targeting Pax7 Decreased Pax7 expression is required to initiate myogenic differentiation [21] . In C2C12 cells, as in SCs ( Fig. 1c ), miR-431 expression was upregulated during differentiation ( Supplementary Fig. 5 ). Since miR-431 targets Pax7 and miR-431 expression correlates negatively with Pax7 expression, miR-431 may regulate myogenic differentiation by modulating Pax7 expression. To investigate this possibility, we stably overexpressed miR-431 or miR-1 (positive control) [29] in C2C12 cells. After confirming the overexpression using real-time reverse-transcription PCR (RT–PCR) ( Supplementary Fig. 6 ), we placed the cells in differentiation medium for 12 and 36 h, respectively, and assayed the expression of two markers of myogenic differentiation: myogenin ( MyoG ) and myosin heavy chain ( MHC ). Myogenic differentiation was stimulated to a much greater extent in cells expressing miR-431 than in negative controls, as shown by the greater abundance of MyoG + ( Fig. 2a ) and MHC + cells ( Fig. 2d ) and by the higher levels of MyoG mRNA ( Fig. 2b ) and protein ( Fig. 2c ) and MHC mRNA ( Fig. 2e ) and protein ( Fig. 2f ). miR-431 and miR-1 enhanced differentiation to a similar extent ( Fig. 2a,d ), revealing that miR-431 regulates myogenic cell differentiation. To determine whether miR-431 does so by targeting Pax7 , we overexpressed Pax7 in C2C12 cells stably expressing miR-431 ( Supplementary Fig. 7 ). Pax7 overexpression abolished the differentiation induced by miR-431, as indicated by the reactivity ( Fig. 2g,h ) and expression ( Fig. 2i ) of MHC. 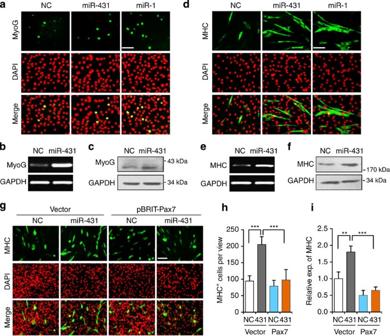Figure 2: miR-431 promotes myogenic differentiation by targetingPax7. (a) The differentiation of C2C12 cells stably overexpressing miR-431 was examined by staining for MyoG after 12 h of culture in DM. Cells overexpressing miR-1 served as the positive control and cells with an empty vector as the NC. Scale bar, 50 μm. (b,c)MyoGexpression in the C2C12 cells described inawas analysed using semiquantitative RT–PCR (b) and western blot analysis (c).GAPDHwas the loading control. (d)The differentiation of C2C12 cells stably overexpressing miR-431 was examined by staining for MHC after 36 h of culture in DM. Cells overexpressing miR-1 served as the positive control and cells with an empty vector as the NC. Scale bar, 50 μm. (e,f) The expression ofMHCin C2C12 cells indwas analysed using semiquantitative RT–PCR (e) and western blot analysis (f).GAPDHwas the loading control. (g) Pax7 was overexpressed in C2C12 cells stably overexpressing miR-431 and NC cells. Differentiation of C2C12 cells was examined by staining for MHC after 24 h of culture in DM. Scale bar, 50 μm. (h) MHC+cells were calculated based on staining described in panelg. (i)MHCexpression in the cells ingdetected using real-time qRT–PCR.GAPDHwas the internal control. Error bars represent means±s.e.m. of three independent experiments. **P<0.01, ***P<0.001. Two-tailed Student’st-test was used for all statistical testing. Figure 2: miR-431 promotes myogenic differentiation by targeting Pax7. ( a ) The differentiation of C2C12 cells stably overexpressing miR-431 was examined by staining for MyoG after 12 h of culture in DM. Cells overexpressing miR-1 served as the positive control and cells with an empty vector as the NC. Scale bar, 50 μm. ( b,c ) MyoG expression in the C2C12 cells described in a was analysed using semiquantitative RT–PCR ( b ) and western blot analysis ( c ). GAPDH was the loading control. ( d )The differentiation of C2C12 cells stably overexpressing miR-431 was examined by staining for MHC after 36 h of culture in DM. Cells overexpressing miR-1 served as the positive control and cells with an empty vector as the NC. Scale bar, 50 μm. ( e,f ) The expression of MHC in C2C12 cells in d was analysed using semiquantitative RT–PCR ( e ) and western blot analysis ( f ). GAPDH was the loading control. ( g ) Pax7 was overexpressed in C2C12 cells stably overexpressing miR-431 and NC cells. Differentiation of C2C12 cells was examined by staining for MHC after 24 h of culture in DM. Scale bar, 50 μm. ( h ) MHC + cells were calculated based on staining described in panel g . ( i ) MHC expression in the cells in g detected using real-time qRT–PCR. GAPDH was the internal control. Error bars represent means±s.e.m. of three independent experiments. ** P <0.01, *** P <0.001. Two-tailed Student’s t -test was used for all statistical testing. Full size image Pax7 Lo SCs are enriched in miR-431 transgenic mice To investigate how the miR-431– Pax7 axis regulates muscle development and regeneration in vivo , we generated two lines of miR-431 transgenic (TG) mice ( Supplementary Fig. 8a ). Real-time RT–PCR analysis showed 4-fold overexpression of miR-431 in the H line and 20-fold overexpression in the O line ( Supplementary Fig. 8b ). Similar to their WT littermates, neither line had histological or overt physiological abnormalities in skeletal muscle during development ( Supplementary Fig. 8c–f ). In skeletal muscle, expression of Pax7 mRNA was significantly lower in both TG mouse lines than in WT littermate controls ( Fig. 3a,b ). The reduced expression did not reflect fewer SCs, which were presented at similar numbers in Pax7-stained muscle sections of WT and TG mice ( Fig. 3c ). 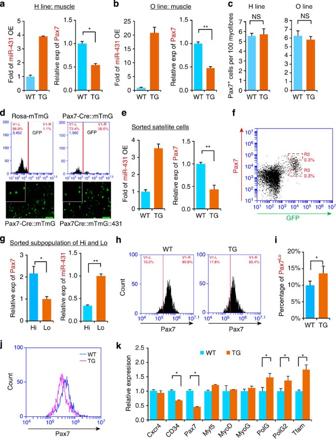Figure 3: Satellite cells in miR-431 TG mice have Pax7Locharacteristics. miR-431 TG mice were generated in which transgene expression was driven by the β-actin promoter (pCAGGS). Two lines of the TG mice (H and O) were used. Values are mean±s.e.m. or one representative value from four to five pairs of WT and TG mice. *P<0.05, **P<0.01. NS, not significant. Two-tailed Student’st-test was used for all statistical testings. (a,b) miR-431 overexpression (OE) levels in the skeletal muscle of the H (a) and O (b) lines were examined using real-time RT–PCR with TaqMan probe. U6 snRNA was the internal control.Pax7expression in the same samples was analysed using real-time RT–PCR andGAPDHwas the internal control. (c) Number of satellite cells in cryosections of TA muscle, stained for Pax7, from miR-431 TG mice and WT controls. (d) Satellite cells were genetically labelled with GFP by crossing miR-431 TG mice withPax7Cre::RosamTmGreporter mice. GFP+cells from the skeletal muscle ofPax7-Cre::RosamTmG::miR-431mice andPax7-Cre::RosamTmGcontrols were sorted using FACS. (e) miR-431 OE in FACS-sorted satellite cells fromdwas determined using real-time RT–PCR. U6 snRNA was the internal control.Pax7expression in the same samples was determined using real-time RT–PCR andGAPDHwas the internal control. (f) Satellite cells sorted from the skeletal muscle ofPax7-Cre::RosamTmGmice were stained with Pax7, and the stained cells were sorted with FACS into Pax7Hiand Pax7Losubpopulations. (g) Expression levels of miR-431 andPax7in the Pax7Hiand Pax7Losatellite cells fromfwere analysed using real-time PCR. (h) Satellite cells were sorted by FACS to select CD31-CD45-Sca1-VCAM+ from miR-431 TG and WT mice and stained with Pax7; the stained satellite cells were further sorted by FACS to calculate Pax7Losubpopulations. (i) The percentage of the Pax7Losubpopulation were calculated based onh,j. Overall profile of Pax7+cells sorted inh,k. Expressions of the stemness-, differentiation- and mitochondria-related markers, determined using real-time RT–PCR in sorted satellite cells from miR-431 TG and WT mice. Figure 3: Satellite cells in miR-431 TG mice have Pax7 Lo characteristics. miR-431 TG mice were generated in which transgene expression was driven by the β-actin promoter (pCAGGS). Two lines of the TG mice (H and O) were used. Values are mean±s.e.m. or one representative value from four to five pairs of WT and TG mice. * P <0.05, ** P <0.01. NS, not significant. Two-tailed Student’s t -test was used for all statistical testings. ( a,b ) miR-431 overexpression (OE) levels in the skeletal muscle of the H ( a ) and O ( b ) lines were examined using real-time RT–PCR with TaqMan probe. U6 snRNA was the internal control. Pax7 expression in the same samples was analysed using real-time RT–PCR and GAPDH was the internal control. ( c ) Number of satellite cells in cryosections of TA muscle, stained for Pax7, from miR-431 TG mice and WT controls. ( d ) Satellite cells were genetically labelled with GFP by crossing miR-431 TG mice with Pax7Cre :: RosamTmG reporter mice. GFP + cells from the skeletal muscle of Pax7-Cre :: RosamTmG :: miR-431 mice and Pax7-Cre :: RosamTmG controls were sorted using FACS. ( e ) miR-431 OE in FACS-sorted satellite cells from d was determined using real-time RT–PCR. U6 snRNA was the internal control. Pax7 expression in the same samples was determined using real-time RT–PCR and GAPDH was the internal control. ( f ) Satellite cells sorted from the skeletal muscle of Pax7-Cre :: RosamTmG mice were stained with Pax7, and the stained cells were sorted with FACS into Pax7 Hi and Pax7 Lo subpopulations. ( g ) Expression levels of miR-431 and Pax7 in the Pax7 Hi and Pax7 Lo satellite cells from f were analysed using real-time PCR. ( h ) Satellite cells were sorted by FACS to select CD31-CD45-Sca1-VCAM+ from miR-431 TG and WT mice and stained with Pax7; the stained satellite cells were further sorted by FACS to calculate Pax7 Lo subpopulations. ( i ) The percentage of the Pax7 Lo subpopulation were calculated based on h , j . Overall profile of Pax7 + cells sorted in h , k . Expressions of the stemness-, differentiation- and mitochondria-related markers, determined using real-time RT–PCR in sorted satellite cells from miR-431 TG and WT mice. Full size image Next, we generated Pax7-Cre :: Rosa26-mTmG :: miR-431 reporter mice and WT controls ( Pax7-Cre :: Rosa26-mTmG ) and isolated green fluorescent protein (GFP)-positive SCs by fluorescence-activated cell sorting (FACS; Fig. 3d ). Despite equal numbers of sorted cells in the two groups, Pax7 expression was remarkably lower in SCs of Pax7-Cre :: Rosa26-mTmG :: miR-431 mice ( Fig. 3e ). Since miR-431 targeted Pax7 in SCs, and TG SCs expressed significantly less Pax7 , we suspected that SCs in miR-431 TG mice are enriched in the Pax7 Lo subpopulation. To directly test this possibility, we examined the expression of endogenous miR-431 and Pax7 in sorted Pax7 Hi and Pax7 Lo SCs from skeletal muscle of Pax7-Cre :: Rosa26-mTmG mice as described [20] ( Fig. 3f ). The miR-431 levels were much lower in Pax7 Hi cells and much higher in the Pax7 Lo cells ( Fig. 3g ). Moreover, the Pax7 Lo subpopulation in sorted cells was increased in TG mice at the expense of decreased Pax7 Hi ( Fig. 3h,i , Supplementary Fig. 9 ). In addition, overexpression of miR-431 shifted the overall profile of SC population towards Pax7 Lo ( Fig. 3j ). Therefore, although there was a 5% increase in Pax7 Lo cells, we did observe the overall twofold Pax7 reduction in the entire population assessed with sensitive quantitative RT–PCR (qRT–PCR; Fig. 3e ). In addition, SCs from TG mice expressed lower levels of Pax7 and stemness-related genes, including C-X-C chemokine receptor type 4 ( CXCR4 ) and cluster of differentiation 34 ( CD34 ), but highly expressed the myogenic differentiation gene MyoG and the mitochondria genes, mitochondrial-specific polymerase γ (catalytic PolG and accessory PolG2 ), and mitochondrial transcription factor A ( Tfam ; Fig. 3k ), which are typical features of Pax7-nGFP Lo cells. Thus, miR-431 TG mice are a potential model system for investigating the biological features of Pax7 Lo cells in vivo . miR-431-mediated Pax7 Lo SCs are primed for differentiation To characterize the function of Pax7 Lo SCs in miR-431 TG mice, we first assessed their myogenic differentiation capability. Freshly isolated SCs from the hindlimb skeletal muscle of TG and WT mice were cultured in the growth medium for 48 h and were immunostained with antibodies against MyoD and MyoG ( Fig. 4a ). MyoD + and MyoG + TG cells were significantly more abundant ( Fig. 4b ), indicating greater myogenic differentiation. Consistently, the differentiation of isolated primary myoblasts was also greater in the TG mice ( Supplementary Fig. 10 ). 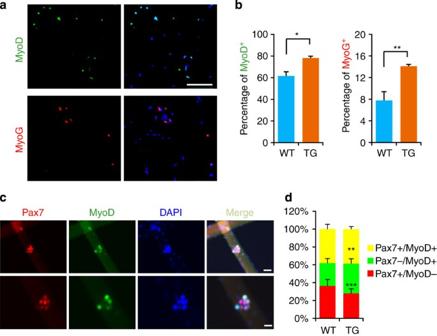Figure 4: Pax7Losatellite cells of miR-431 TG mice are more primed for differentiation than the WT controls. (a) Satellite cells from thePax7Cre::R26mTmG::miR-431and Pax7Cre::R26mTmGcontrols were sorted using FACS, cultured for 48 h in growth medium and immunostained for MyoD (green) and MyoG (red). Blue, 4′,6-diamidino-2-phenylindole dihydrochloride (DAPI) staining. Scale bars, 100 μm. (b) Numbers of the MyoD+ and MyoG+ cells ina. Values are means±s.e.m. of triplicate experiments. *P<0.05, **P<0.01. Two-tailed Student’st-test was used for all statistical testings. (c) Double staining for Pax7 and MyoD in expanded satellite cells from single fibres isolated from EDL muscle and cultured for 72 h. The data are from five mice for each genotype and more than 200 myofibres were analysed. Scale bar, 50 μm. (d) Numbers of Pax7+/MyoD+, Pax7–/MyoD+and Pax7+/MyoD–cells in cultured single fibres from miR-431 TG and WT mice inc. Values are means±s.e.m. **P<0.01, ***P< 0.001. Two-tailed Student’st-test was used for all statistical testings. Figure 4: Pax7 Lo satellite cells of miR-431 TG mice are more primed for differentiation than the WT controls. ( a ) Satellite cells from the Pax7Cre :: R26mTmG :: miR-431 and Pax7Cre:: R26mTmG controls were sorted using FACS, cultured for 48 h in growth medium and immunostained for MyoD (green) and MyoG (red). Blue, 4′,6-diamidino-2-phenylindole dihydrochloride (DAPI) staining. Scale bars, 100 μm. ( b ) Numbers of the MyoD+ and MyoG+ cells in a . Values are means±s.e.m. of triplicate experiments. * P <0.05, ** P <0.01. Two-tailed Student’s t -test was used for all statistical testings. ( c ) Double staining for Pax7 and MyoD in expanded satellite cells from single fibres isolated from EDL muscle and cultured for 72 h. The data are from five mice for each genotype and more than 200 myofibres were analysed. Scale bar, 50 μm. ( d ) Numbers of Pax7 + /MyoD + , Pax7 – /MyoD + and Pax7 + /MyoD – cells in cultured single fibres from miR-431 TG and WT mice in c . Values are means±s.e.m. ** P <0.01, *** P < 0.001. Two-tailed Student’s t -test was used for all statistical testings. Full size image Next, we investigated the differentiation and self-renewal of SCs—which must be precisely balanced to maintain muscle tissue homeostasis during normal development and regeneration—in myofibre-associated SCs. In single fibres isolated from extensor digitorum longus (EDL) muscle and cultured ex vivo for 72 h, immunostaining showed the typical clusters of SC progeny that are proliferating (Pax7 + /MyoD + ), differentiating (Pax7 – /MyoD + ) and self-renewing (Pax7 + /MyoD – ; Fig. 4c ). However, miR-431 TG myofibres had significantly more differentiating cells and significantly fewer self-renewing cells than WT controls ( Fig. 4d ), indicating precocious onset of differentiation in the TG cells. Together, our ex vivo and in vivo data convincingly suggest that miR-431 TG mice are enriched in Pax7 Lo SCs that are primed more for differentiation and less for self-renewal. Muscle regeneration is accelerated in miR-431 TG mice Since miR-431 targets Pax7 and promotes muscle cell differentiation in vitro , we next investigated how it regulates SC function during muscle regeneration. Muscle regeneration was induced by injecting cardiotoxin (CTX) into tibialis anterior (TA) muscle of WT and miR-431 TG mice of lines O and H. Similar results were obtained in both TG lines; therefore, we present data from the H line. During regeneration, miR-431 expression dropped immediately in response to injury after CTX injection ( Supplementary Fig. 11 ), consistent with the greater downregulation of miR-431 in activated than in quiescent SCs [27] . Myogenic differentiation happens within 3 days post injury during muscle regeneration; we indeed observed increased expression of miR-431 at 3 days and it was remarkably elevated after the time point ( Supplementary Fig. 11 ). This expression pattern suggests that miR-431 helps to mediate SC function during regeneration of damaged muscle. In support of this notion, at 7 days after injection, regenerating myofibres, characterized by centralized nuclei, were significantly larger in miR-431 TG mice than in WT controls ( Fig. 5a,b ). 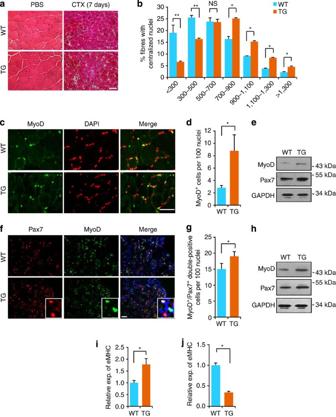Figure 5: miR-431 TG mice exhibit accelerated skeletal muscle regeneration. The H and O lines of the miR-431 TG mice had similar phenotypes. The data presented here are from the analysis of H line mice. Values are mean±s.e.m. or one representative value from five pairs of WT and TG mice. *P<0.05, **P<0.01. NS, not significant. Two-tailed Student’st-test was used for all statistical testings. (a) Representative haematoxylin and eosin (H&E)-stained sections of TA muscle 7 days after injury induced by CTX injection. Controls were injected with PBS. Scale bar, 50 μm. (b) Cross-sectional area of regenerated myofibres with centralized nuclei, calculated from the H&E-stained sections ina,c. A representative view of MyoD staining on sections of TA muscle 1 day after CTX injury. Green, MyoD; red, DAPI. Scale bar, 50 μm. (d) Number of MyoD+cells in sections of TA muscle 1 day after CTX injury (shown inc). (e) Western blots showing expression levels of MyoD and Pax7 in TA muscle 1 day after CTX injury. GAPDH was the loading control. (f) Representative sections of TA muscle 3 days after CTX injury, double-stained for Pax7 (red) and MyoD (green). Scale bar, 50 μm. (g) Number of Pax7+/MyoD+double-positive cells in sections of TA muscle 3 days after CTX injury (shown inf). (h) Western blots showing expression of MyoD and Pax7 in TA muscle 3 days after CTX injury. GAPDH was the loading control. (i,j) Expression ofeMHCin TA muscle 3 days (i) and 7 days (j) after injury, detected using RT–qPCR. Figure 5: miR-431 TG mice exhibit accelerated skeletal muscle regeneration. The H and O lines of the miR-431 TG mice had similar phenotypes. The data presented here are from the analysis of H line mice. Values are mean±s.e.m. or one representative value from five pairs of WT and TG mice. * P <0.05, ** P <0.01. NS, not significant. Two-tailed Student’s t -test was used for all statistical testings. ( a ) Representative haematoxylin and eosin (H&E)-stained sections of TA muscle 7 days after injury induced by CTX injection. Controls were injected with PBS. Scale bar, 50 μm. ( b ) Cross-sectional area of regenerated myofibres with centralized nuclei, calculated from the H&E-stained sections in a , c . A representative view of MyoD staining on sections of TA muscle 1 day after CTX injury. Green, MyoD; red, DAPI. Scale bar, 50 μm. ( d ) Number of MyoD + cells in sections of TA muscle 1 day after CTX injury (shown in c ). ( e ) Western blots showing expression levels of MyoD and Pax7 in TA muscle 1 day after CTX injury. GAPDH was the loading control. ( f ) Representative sections of TA muscle 3 days after CTX injury, double-stained for Pax7 (red) and MyoD (green). Scale bar, 50 μm. ( g ) Number of Pax7 + /MyoD + double-positive cells in sections of TA muscle 3 days after CTX injury (shown in f ). ( h ) Western blots showing expression of MyoD and Pax7 in TA muscle 3 days after CTX injury. GAPDH was the loading control. ( i,j ) Expression of eMHC in TA muscle 3 days ( i ) and 7 days ( j ) after injury, detected using RT–qPCR. Full size image Next, to evaluate the influence of miR-431 on SC activation, proliferation and differentiation during regeneration, we immunostained sections with antibodies against Pax7 and MyoD ( Fig. 5c,f ). Pax7 is expressed in quiescent and activated SCs, and MyoD is expressed in SCs that are activated during muscle regeneration [10] , [35] , [36] . At 1 day after CTX injection, MyoD + cells were more numerous in TG mice ( Fig. 5d ) and MyoD protein was more abundant in TG muscle ( Fig. 5e ). Thus, miR-431 promoted SC activation early on during muscle regeneration. Moreover, at 3 days after injection, TG mice also had more Pax7 + and MyoD + cells ( Fig. 5f,g ) and more Pax7 and MyoD proteins ( Fig. 5h ), indicating that miR-431 caused activated SCs to proliferate during the proliferative phase of muscle regeneration. At 3 days, the well-defined myogenic differentiation marker MHC 3 ( Myh3 ), also called embryonic MHC ( eMHC ), was highly expressed in the damaged muscle of TG mice but not of WT mice ( Fig. 5i ), indicating precocious differentiation in miR-431 TG mice. At 7 days after injection, Myh3 mRNA was less abundant in the damaged muscles of the TG mice than that of WT mice ( Fig. 5j ), showing that neonatal myofibres formed faster in TG mice than in WT controls. At 31 days after CTX injection, the number of Pax7 + cells ( Fig. 6a,b ) and the levels of Pax7 protein ( Fig. 6c ) and mRNA ( Fig. 6d ) were significantly lower in TG mice, whereas MyoG mRNA levels in muscle ( Fig. 6e ) were much higher. Thus, miR-431 overexpression has a long-term functional effect in promoting the muscle regeneration in mice. 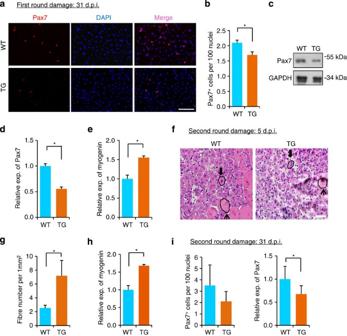Figure 6: miR-431 does not deplete the satellite pool after two rounds of injury. One representative value or means±s.e.m. from five pairs of WT and TG mice. *P<0.05. Two-tailed Student’st-test was used for all statistical testings. (a) Pax7 staining on sections of CTX-damaged TA muscles from miR-431 TG and WT mice 31 days after injury (d.p.i.). Scale bar, 50 μm. (b) Number of Pax7-positive cells in the stained sections ina. (c) Western blots showing Pax7 expression in injured TA muscle 31 d.p.i. (d,e)Pax7and myogenin gene expression in the samples incwere determined using real-time RT–PCR.GAPDHwas the internal control. (f) Newly formed regenerated myofibres with centralized nuclei in H&E-stained sections of TA muscle 5 days after the second round of CTX injury. Scale bar, 50 μm. (g) Numbers of regenerated myofibres in sections inf,h.MyoGgene expression in the samples inf, analysed using real-time RT–PCR.GAPDHwas the internal control. (i) Number of Pax7-positive cells in sections of TA muscle at 31 days after the second round of CTX-induced injury. Pax7 expression in the same samples was examined using real-time RT–PCR. Figure 6: miR-431 does not deplete the satellite pool after two rounds of injury. One representative value or means±s.e.m. from five pairs of WT and TG mice. * P <0.05. Two-tailed Student’s t -test was used for all statistical testings. ( a ) Pax7 staining on sections of CTX-damaged TA muscles from miR-431 TG and WT mice 31 days after injury (d.p.i.). Scale bar, 50 μm. ( b ) Number of Pax7-positive cells in the stained sections in a . ( c ) Western blots showing Pax7 expression in injured TA muscle 31 d.p.i. ( d,e ) Pax7 and myogenin gene expression in the samples in c were determined using real-time RT–PCR. GAPDH was the internal control. ( f ) Newly formed regenerated myofibres with centralized nuclei in H&E-stained sections of TA muscle 5 days after the second round of CTX injury. Scale bar, 50 μm. ( g ) Numbers of regenerated myofibres in sections in f,h . MyoG gene expression in the samples in f , analysed using real-time RT–PCR. GAPDH was the internal control. ( i ) Number of Pax7-positive cells in sections of TA muscle at 31 days after the second round of CTX-induced injury. Pax7 expression in the same samples was examined using real-time RT–PCR. Full size image Since TG SCs were preferentially differentiated rather than self-renewed, we thought that TG mice subjected to a second CTX-induced injury might have fewer quiescent SCs and an increased number of smaller myofibres than WT mice. Indeed, 5 days after the second injury, TG mice had smaller myofibres in greater abundance ( Fig. 6f,g ) and higher levels of MyoG mRNA ( Fig. 6h ) in newly formed regenerated myofibres. Moreover, at 31 days, TG mice had no change in the number of Pax7 + SCs, but Pax7 transcripts were significantly lower than those in WT mice ( Fig. 6i ). The morphological and molecular evidence supports the notion that myogenic differentiation is remarkably accelerated in miR-431 TG mice during muscle regeneration. Although we have noticed that MyoD expression in the SCs of damaged muscle ( Fig. 5g ) from TG mice was inconsistent with that of ex vivo cultured single fibres ( Fig. 4d ), it is possible that the inconsistence might be due to the different responses of SCs under the two experimental conditions. Together, our findings indicate that miR-431 may help to accelerate muscle regeneration in mice by mediating SC functions with enriched subpopulation of Pax7 Lo SCs, which are primed more for differentiation and less for self-renewal. The miR-431 transgene reduces muscular dystrophy in mdx mice Since miR-431 accelerated muscle regeneration in mice, we investigated the possibility that it would reduce muscular dystrophy in mice. We generated mdx mice overexpressing miR-431 ( miR-431 :: mdx ; Supplementary Fig. 12 ) and compared their muscular morphology with that of mdx mice. The two groups of mice did not differ overtly in muscle mass, muscle architecture or the number and size of myofibres ( Supplementary Fig. 13 ). To further characterize the dystrophic phenotype of miR-431 :: mdx mice, we measured serum creatine kinase levels, an indicator of skeletal muscle damage, and examined membrane permeability of myofibres by their uptake of Evans blue dye [37] . Serum creatine kinase levels were 12-fold higher in mdx mice than in WT mice (C57BL/6 mice), but were significantly lower in miR-431 :: mdx than in mdx mice ( Fig. 7a ). The Evans blue dye uptake was also significantly lower in miR-431 :: mdx than in mdx mice ( Fig. 7b,c ). These morphological findings indicate that miR-431 overexpression reduces the dystrophic phenotype of mdx mice. 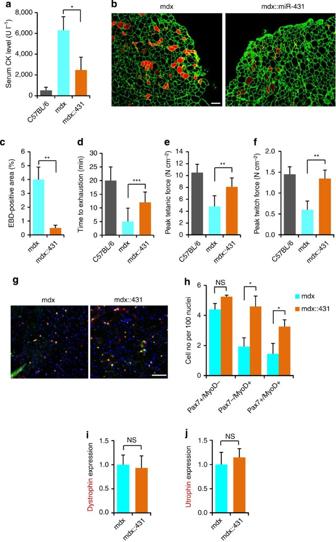Figure 7: The miR-431 transgene reduces the dystrophic phenotype inmdxmice. miR-431::mdxmice were generated by crossing miR-431 TG mice withmdxmice. Values are means±s.e.m. of experiments with five to eight mice at 5 months of age.*P<0.05, **P<0.01, ***P<0.001. NS, not significant. (a) Serum creatine kinase (CK) levels in C57BL/6 WT andmdxcontrol ormiR-431::mdxmice. (b) Evans blue dye uptake in TA muscle. Scale bar, 50 μm. (c) Percentage of Evans blue-positive fibre area in TA muscle ofmdxandmiR-431::mdxmice. (d) Running time to exhaustion on the downhill treadmill test. (e) Maximal twitch force induced by electrical stimulationin vitroto elicit tetanic contractions in EDL muscle from C57BL/6,mdxandmiR-431::mdxmice. (f) Peak twitch force induced in EDL muscle by electrical stimulationin vitro. (g) Pax7 (red) and MyoD (green) double staining on sections of TA muscles frommdxandmdx::miR-431mice. Scale bar, 100 μm. (h) Numbers of Pax7+/MyoD+, Pax7–/MyoD+and Pax7+/MyoD–cells in the stained sections ing. (i,j) Expression of dystrophin (i) and utrophin (j) in TA muscle of mdx andmdx::miR-431mice, analysed using real-time RT–PCR.GAPDHwas the internal control. Figure 7: The miR-431 transgene reduces the dystrophic phenotype in mdx mice. miR-431 :: mdx mice were generated by crossing miR-431 TG mice with mdx mice. Values are means±s.e.m. of experiments with five to eight mice at 5 months of age. * P <0.05, ** P <0.01, *** P <0.001. NS, not significant. ( a ) Serum creatine kinase (CK) levels in C57BL/6 WT and mdx control or miR-431 :: mdx mice. ( b ) Evans blue dye uptake in TA muscle. Scale bar, 50 μm. ( c ) Percentage of Evans blue-positive fibre area in TA muscle of mdx and miR-431 :: mdx mice. ( d ) Running time to exhaustion on the downhill treadmill test. ( e ) Maximal twitch force induced by electrical stimulation in vitro to elicit tetanic contractions in EDL muscle from C57BL/6, mdx and miR-431 :: mdx mice. ( f ) Peak twitch force induced in EDL muscle by electrical stimulation in vitro . ( g ) Pax7 (red) and MyoD (green) double staining on sections of TA muscles from mdx and mdx :: miR-431 mice. Scale bar, 100 μm. ( h ) Numbers of Pax7 + /MyoD + , Pax7 – /MyoD + and Pax7 + /MyoD – cells in the stained sections in g . ( i,j ) Expression of dystrophin ( i ) and utrophin ( j ) in TA muscle of mdx and mdx :: miR-431 mice, analysed using real-time RT–PCR. GAPDH was the internal control. Full size image To assess muscle function and performance in the mice, we measured running time to exhaustion in a downhill treadmill exercise paradigm. At 5 months of age, mdx mice ran for a significantly shorter time than WT controls (C57BL/6 mice; Fig. 7d ). However, miR-431 :: mdx mice had longer running times compared with mdx mice, indicating less muscle injury and less dysfunction. In addition, the peak tetanic force was 2.5-fold greater ( Fig. 7e ) and the peak twitch force was 3-fold greater ( Fig. 7f ) in miR-43 1:: mdx mice. To further confirm that miR-431 regulates SC proliferation and differentiation during the degeneration/regeneration cycle, we immunostained SCs in sections of regenerating TA muscle with antibodies against Pax7 and MyoD ( Fig. 7g ). Proliferating (Pax7 + /MyoD + ) and differentiating (Pax7 – /MyoD + ) cells were significantly more abundant in mdx :: miR-431 muscle than in mdx muscle ( Fig. 7h ), further corroborating the critical role of miR-431 in promoting proliferation and differentiation of activated SCs during skeletal muscle regeneration in mice. Since the miR-431 transgene driven by the chicken β-actin promoter was also overexpressed in myofibres of the TG mice, miR-431 might improve the dystrophic phenotype in mdx mice by direct effects on myofibre structure and function. To test this possibility, we examined expression of dystrophin and utrophin ( Fig. 7i,j ) and gene markers of different types of myofibres ( Supplementary Fig. 14a ) and genes related to the metabolic features of the fibre types ( Supplementary Fig. 14b ) in the TA muscle. The tested genes were expressed at similar levels in mdx :: 431 and mdx mice. Evidently, miR-431 reduces muscular dystrophy in mdx :: miR-431 mice mainly through effects on SC functions. Overall, these findings are consistent with the histological and morphological data and suggest a molecular explanation of how miR-431 overexpression functionally reduces the dystrophic phenotype in mdx mice. The functional relevance of SC heterogeneity is illustrated by the distinct myogenic and metabolic features of Pax7 Hi and Pax7 Lo SCs [20] . For example, Pax7 Lo cells are more committed to myogenic differentiation than the stem-like Pax7 Hi cells [20] . It has been reported that Pax7 Hi and Pax7 Lo subpopulations are mediated at the transcriptional level [20] . However, how is the level of Pax7 post-transcriptionally regulated in SCs to establish these different subpopulations, and what biological effects do these subpopulations have in vivo ? In this study, we showed that miR-431 is predominantly expressed in the skeletal muscle and post-transcriptionally fine-tunes the Pax7 level by directly targeting Pax7 in SCs. Significantly, we found that Pax7 Lo SCs are remarkably enriched in miR-431 TG mice, indicating that miR-431 has a critical role in controlling SC heterogeneity by mediating the Pax7 level. Furthermore, we found that Pax7 Lo cells have a greater potential for myogenic differentiation and, in miR-431 TG mice, they speed muscle regeneration by promoting SC differentiation. Finally, we found that overexpression of miR-431 in a mouse model of muscular dystrophy ( miR-431 : :mdx mice) markedly reduces the disease phenotype. miR-431 is from the miRNA cluster that is processed from the antisense strand of maternally expressed imprinted gene Rtl1 (ref. 38 ). Rtl1 is a paternally expressed intronless protein-coding gene, and six miRNAs (miR-431, miR-433, miR-127, miR-434, miR-432 and miR-136) are maternally generated when the Rtl1 gene is transcribed in the opposite direction [39] , [40] , [41] . However, until now, no evidence has indicated the function of these miRNAs in muscle development and regeneration. We showed that miR-431 is predominantly expressed in the skeletal muscle and regulates myogenesis in vitro and in vivo by targeting Pax7 . Other studies suggested that miRNAs from the anti-Rtl1 strand directly target Rtl1 , causing the Rtl1 transcript to be cleaved by the RNA-induced silencing complex [40] . Still other studies suggested that Rtl1 is associated with the double-muscled phenotype of Callipyge sheep ( CLPG region) [39] , suggesting that this genetic locus helps to regulate muscle development and regeneration. However, we found no difference in Rtl1 expression in the skeletal muscle of miR-431 TG and WT control mice ( Supplementary Fig. 15 ). Thus, miR-431 regulates myogenic differentiation independently of Rtl1 . We used several strategies to show that miR-431 TG muscle harbours more Pax7 Lo SCs, which are prone to be more primed for differentiation in response to myogenic stimuli. Pax7 expression was lower in SCs from TG mice than in those from WT controls. Moreover, the biological features of SCs from miR-431 TG mice were very similar to those reported for Pax7 Lo cells [27] . First, SCs from miR-431 TG mice had fewer stemness markers ( CXCR4 and CD34 ) and higher expression of the differentiation gene MyoG . Second, SCs from TG mice more readily underwent differentiation and less readily underwent self-renewal. Our findings reveal a critical role for miR-431 in establishing and maintaining SC heterogeneity by fine-tuning Pax7 expression, and they provide a novel mechanism for generating mice with an enhanced population of Pax7 Lo SCs. Pax7 is a key regulator of SC proliferation, self-renewal and differentiation, and its expression and transcriptional activity are tightly regulated. For example, MyoG represses Pax7 transcription by binding to regulatory sequences in the Pax7 promoter via the HMGB1–RAGE axis. Rage –/– myoblasts have higher levels of Pax7, greater proliferation potential and lower differentiation potential than WT myoblasts, and deleting Rage promotes asymmetric division of myoblasts [42] . MyoD and MyoG downregulate Pax7 post-translationally [43] ; however, in myoblasts committed to differentiation, post-transcriptional downregulation is mediated by miR-1, miR-206 and miR-486 (refs 30 , 44 ). Here we showed that miR-431 regulates SC functions in miR-431 TG mice and we provide convincing evidence that the Pax7 level is tightly controlled by miR-431 in SCs in vitro and in vivo . Furthermore, we found that miR-431 critically regulates the establishment and maintenance of the Pax7 Lo subpopulation in mice by targeting Pax7 . More intriguingly, cells in the Pax7 Lo subpopulation described in ref. 20 have a higher metabolic status, as shown by their higher ATP levels and better oxidative capacity. However, the functional relevance of this specific and unique feature of Pax7 Lo cells has not been explored yet, and fundamental questions remain to be addressed. Why and how are the metabolic features of the Pax7 Lo subpopulation correlated to biological processes during skeletal muscle development and regeneration? What molecular mechanism underlies the metabolic state of Pax7 Lo cells? Our miR-431 TG mice, which harbour an enriched Pax7 Lo subpopulation, will be a good genetic model for answering these questions about skeletal muscle development and regeneration. Finally, we also showed that in mdx mice, a model of Duchenne muscular dystrophy [45] , miR-431 lessens the severity of the phenotype. Although this disease is caused primarily by a mutation in the gene encoding dystrophin [46] , several genes slow disease progression in mdx mice [47] , [48] , [49] , [50] . Thus, therapeutic strategies may not be limited to those directly targeting the dystrophin gene. Interestingly, many studies suggest that the genes controlling SC proliferation and differentiation strongly influence the pathogenesis of mdx mice. For example, Wnt7a ameliorates muscular dystrophy in mdx mice by stimulating SC expansion and myofibre hypertrophy via the AKT/mTOR anabolic pathway [51] . Moreover, miR-206 delays the progression of muscular dystrophy in mdx mice by promoting SC differentiation through targeting negative regulators of myogenic differentiation, including Notch3 , Pax7 and IGFbp5 (ref. 52 ). Our finding that miR-431 markedly reduces the dystrophic phenotype in miR-431 :: mdx mice raises the possibility that delivering miR-431 mimics or manipulating the downstream targets of miR-431 will benefit patients with Duchenne muscular dystrophy (DMD) or other muscular diseases. Mice and animal care All animal procedures were approved by the Animal Ethics Committee of Peking Union Medical College, Beijing, China. Mice were housed in the animal facility and had free access to water and standard rodent chow. miR-431 TG mice were generated by the Model Animal Research Center of the Nanjing University. Rosa26-mTmG mice were a gift from Dr Shihuan Kuang (Purdue University). Mdx mice were from the Model Animal Research Center of the Nanjing University. Pax7-Cre mice were provided by Dr Zhenguo Wu (The Hong Kong University of Science and Technology). C57BL/6 mice were purchased from the Vital River Laboratories Company in Beijing. Cell sorting SCs were FACS-sorted from different mouse lines, including miR-431 TG and WT mice and Pax7-Cre :: Rosa26-mTmG :: miR-431 TG and Pax7-Cre :: Rosa26-mTmG male reporter mice at 4 weeks. Mononucleated muscle-derived cells were isolated from hindlimb muscles using dispase and collagenase digestion. The cells from the two reporter cell lines were directly sorted with a BD Aria II Cell Sorting System. Mononuclear cells from non-reporter mice were blocked with goat serum for 10 min and were incubated with antibodies against CD45, CD31, Sca1 and VCAM in DMEM with 2% fetal bovine serum (FBS) for 15 min at 4 °C. Antibodies used to sort SCs include FITC-CD45 (553080, 1:100 dilution), FITC-CD31 (553372, 1:100 dilution), PE-Sca1 (553108, 1:100 dilution), biotin-VCAM (553331, 1:100 dilution) and streptavidin-APC (554067, 1:100 dilution; all from BD Pharmingen). Immunostained cells were briefly washed, passed through a 40-μm nylon mesh (Falcon) and suspended at a concentration of 10 3 –10 7 cells per ml. Cells were further separated with the BD Aria II. Sorting gates were strictly defined on the basis of control cells stained with single antibodies as well as the patterns of forward scatter and side scatter of SCs in preliminary tests. Muscle injury and regeneration Muscle regeneration was induced by injections of CTX (Sigma). Male mice at 8 weeks were anaesthetized by intraperitoneal injection of ketamine (10 mg kg −1 ) and xylazine (1 mg kg −1 ) For monitoring muscle regeneration, muscle injury was induced in 8-week-old mice by injecting CTX (50 μl of 10 μM CTX in PBS) into the midbelly of the right TA muscle. As an internal control, the left TA muscle of each mouse was injected with PBS (50 μl). Muscles were harvested at 1, 3, 5 and 7 days after injection to assess the completion of regeneration and repair. Cell culture C2C12 cells were cultured in the growth medium consisting of DMEM (Gibco) supplemented with 4.5 g l −1 glucose, 10% FBS, 1% antibiotic/antimycotic and 1% gentamycin at 37 °C in a 5% CO 2 atmosphere. At 50–60% confluence, cells were switched to differentiation medium (DMEM with 2% horse serum). C2C12 cell lines stably overexpressing miR-431 were established by infection with lentivirus containing H1-miR-431-CMV-Puromycin (Genechem). Pax7 overexpression plasmids were a gift from Dr Denis C. Guttridge (The Ohio State University). Isolating and staining single myofibres Single myofibres were isolated from the EDL muscles of 8-week-old male mice by digestion with collagenase I (C-0130, Sigma). The muscle was incubated in 3 ml of 0.2% collagenase I in serum-free DMEM in a shaking water bath at 37 °C for 45–60 min. Digestion was considered complete when the muscle looked less defined and slightly swollen, with hair-like single fibres flowing away from the edges. The digested muscles were placed in a Petri dish, and myofibres were isolated under a microscope. Single fibres were placed in six-well plates pre-coated with horse serum. Then, 2 ml of fibre medium (DMEM supplemented with 20% FBS, 0.5% chick embryo extract and penicillin–streptomycin) was added. The fibres were cultured for 72 h at 37 °C in a 5% CO 2 atmosphere, fixed with 4% paraformaldehyde and stained for Pax7 and MyoD. For statistical analyses, Pax7 + and MyoD – cells were counted in at least 40 single fibres per mouse in five pairs of TG and WT mice. Isolating primary myoblasts Primary myoblasts were isolated from the hindlimb skeletal muscle of male mice at 4 weeks, minced and digested in a mixture of type I collagenase and Dispase B (Roche Applied Science). Cells were filtered from debris, centrifuged and cultured in growth medium (F-10 Ham’s medium supplemented with 20% FBS, 4 ng ml −1 basic fibroblast growth factor and 1% penicillin–streptomycin) on collagen-coated cell culture plates at 37 °C in 5% CO 2 (ref. 53 ). Northern blot analysis Total RNA was extracted from the heart, liver, brain, lung, kidney, intestine, spleen and skeletal muscle of 3-week-old male mice, separated using PAGE (7 M urea) on 15% gels, and transferred to a nylon membrane (N+; Amersham). T4 DNA kinase (Fermentas) was used to label miR-431 probes with γ- 32 p-ATP. RNA blots were hybridized in ULTRAhyb (Ambion) at 42 °C overnight, washed twice (5 min each) with 2 × SSC/0.1% SDS wash buffer at 42 °C, followed by stringent washes (2 × 30 min) with 0.1 × SSC/0.1% SDS wash buffer at 42 °C. RNA blots were then exposed to X-ray film at −80 °C. Full scans of northern blots were presented in Supplementary Fig. 16 . Western blot analysis Muscle tissues and C2C12 cells were lysed in a buffer containing 50 mM Tris pH 7.5, 150 mM NaCl, 0.5% Nonidet P40 and protease and phosphatase inhibitors. The protein lysates were resolved using SDS–PAGE, transferred to a polyvinylidene fluoride membrane and immunoblotted with primary antibodies against MHC (MF20, 1:500), MyoG (F5D, 1:500) and Pax7 (from DSHB, 1:500); MyoD (BD Biosciences, 1:250); and GAPDH (Glyceraldehyde 3-phosphate dehydrogenase; Millipore, 1:10,000). Membranes were washed for 30 min, incubated with horseradish peroxidase-conjugated secondary antibodies (Zhongshanjinqiao Corporation) for 1 h at room temperature and washed for 30 min. Each membrane was then placed into Detection Solution (Thermo), incubated for 1 min at room temperature and exposed to X-ray film. Full scans of all western blots are available in Supplementary Fig. 17 . Immunohistochemistry C2C12 cells were seeded in 12-well plates (1 × 10 4 cells per cm 2 per well) in the growth medium; at 50–60% confluence, the cells were transferred to the differentiation medium for 24 or 36 h, fixed with 4% formaldehyde for 5 min and permeabilized in 0.1% Triton X-100 in PBS for 15 min at room temperature. Cells were blocked with 3% bovine serum albumin for 30 min and then incubated with primary antibodies (F5D, 1:200; MF20, 1:300) for 1 h. Fluorescein-conjugated anti-mouse secondary antibodies (Zhongshanjinqiao Corporation; 1:200) were added in 0.1% Triton X-100 plus 3% bovine serum albumin in PBS for 1 h at 37 °C. 4′,6-diamidino-2-phenylindole dihydrochloride was then added for 2 min at room temperature. After several washes with PBS, cells were examined using fluorescence microscopy. RT–PCR and real-time RT–PCR analyses Total RNA from cells was extracted with Trizol reagent (Invitrogen). Expression of mature miRNAs was determined with the miRNA-specific TaqMan microRNA assay kit (Applied Biosystems) and the ABI IQ5 Sequence Detection System (Applied Biosystems). U6 was used for normalization. mRNA expression was analysed with Fast EvaGreenqPCR Master Mix (Applied Biosystems) and normalized to GAPDH. All primers used for RT–PCR were included in Supplementary Table 1 . Transfection and luciferase assays For construction of the 3′-UTR-luciferase reporter, the multiple cloning site of the pGL-3-Control vector (Promega) was removed and placed downstream of the luciferase gene. The 3′-UTRs of mouse Pax7 were amplified using PCR and were cloned into the pGL-3-Control vector, resulting in Pax7-3′-UTR constructs. HEK 293 cells were co-transfected with Pax7-3′-UTR and miR-431 mimics. Empty pGL-3 vector was a negative control. w-UTR is a Pax7 -3′-UTR with miR-431-binding site inserted downstream of the luciferase gene in the pGL-3 control vector. m1utr and m2utr are mutant forms of the Pax7 3′-UTR. A Renilla luciferase plasmid was co-transfected with a firefly luciferase construct as a transfection control. The results are expressed as firefly luciferase activity relative to Renilla luciferase activity. Treadmill The treadmill test was performed using the Exer3/6 (Columbus Instruments). Mice were acclimated to treadmill running four times (every other day) before the test. Mice ran on the treadmill at 20° downhill, starting at a speed of 16 cm s −1 . After 3 min, the speed was increased by 2 cm s −1 to a final speed of 36 cm s −1 . Exhaustion was defined as the inability of the mouse to remain on the treadmill, despite electrical prodding. Force measurements EDL muscles were constantly immersed in physiological saline solution containing 118.5 mM NaCl, 4.7 mM KCl, 2.4 mM CaCl 2 , 3.1 mM MgCl 2 , 25 mM NaHCO 3 , 2 mM NaH 2 PO 4 and 5.5 mM D-glucose. All solutions were continuously bubbled with 95% O 2 /5% CO 2 (vol/vol) and maintained at pH 7.4. All experiments were carried out at 25 °C. Contractions were elicited by passing a current between two platinum electrodes placed on opposite sides of the muscle. Twitch contractions were elicited with a single 0.3-ms square pulse of 10 V (supramaximal voltage); tetanic contractions were elicited with a 200-ms train of the same pulse at 200 Hz. Contractions were elicited every 2 min during the experiment. Muscle length was adjusted to obtain maximum tetanic force, and a 30-min equilibrium period was allowed before force–frequency measurements. Force was measured with a dual-mode muscle lever system (Grass X88 Stimulator) and digitized at 5 kHz with a analogue-digital board (Grass). Peak twitch force and peak tetanic force were calculated as the difference between the maximum force during contraction and the force measured at 5 ms before the contraction. Statistical analysis Values are presented as means±s.e.m. The statistical significance of the difference between two the means was calculated with the t -test. P <0.05 was considered statistically significant. How to cite this article: Wu, R. et al . MicroRNA-431 accelerates muscle regeneration and ameliorates muscular dystrophy by targeting Pax7 in mice. Nat. Commun. 6:7713 doi: 10.1038/ncomms8713 (2015).